Metabotropic P2Y1 receptor signalling mediates astrocytic hyperactivityin vivoin an Alzheimer’s disease mouse model Astrocytic network alterations have been reported in Alzheimer’s disease (AD), but the underlying pathways have remained undefined. Here we measure astrocytic calcium, cerebral blood flow and amyloid-β plaques in vivo in a mouse model of AD using multiphoton microscopy. We find that astrocytic hyperactivity, consisting of single-cell transients and calcium waves, is most pronounced in reactive astrogliosis around plaques and is sometimes associated with local blood flow changes. We show that astroglial hyperactivity is reduced after P2 purinoreceptor blockade or nucleotide release through connexin hemichannels, but is augmented by increasing cortical ADP concentration. P2X receptor blockade has no effect, but inhibition of P2Y1 receptors, which are strongly expressed by reactive astrocytes surrounding plaques, completely normalizes astrocytic hyperactivity. Our data suggest that astroglial network dysfunction is mediated by purinergic signalling in reactive astrocytes, and that intervention aimed at P2Y1 receptors or hemichannel-mediated nucleotide release may help ameliorate network dysfunction in AD. Alzheimer’s disease (AD) is a common and incurable neurodegenerative disease characterized by severe and progressive loss of memory and cognitive function. Formation of toxic amyloid-β (Aβ) species and their accumulation in plaques are key steps in the pathogenesis of AD [1] . The precise mechanisms leading to neurodegeneration in AD are incompletely understood, but are probably related to a multifactorial interplay between direct neurotoxicity, cerebrovascular pathology, inflammation and cortical network dysfunction [1] , [2] , [3] . Glia are arguably the most important safeguards of neuronal health. Astrocytes, in particular, support synaptic function and plasticity, provide energy substrates and contribute to the regulation of regional cerebral blood flow (CBF) [4] , [5] . In essentially every neurological disease, astrocytes change morphologically to adopt a ‘reactive’ phenotype [6] . Reactive astrogliosis represents a universal defence mechanism of the brain to acute and chronic injury, and is also an early and very prominent feature of AD [7] , [8] . Reactive astrogliosis first becomes apparent in the vicinity of nascent Aβ plaques [7] and progresses as plaque load increases. However, it has largely remained undefined how morphological changes in astrocytes translate into functional alterations. This question is particularly important, as most brain functions supported by astrocytes—synaptic health and plasticity, cerebrovascular regulation, inflammatory reactions and network homoeostasis—are also critically impaired in AD, suggesting that a better understanding of astrocyte dysfunction may ultimately lead to novel treatment options in AD. Recently, it was found that astrocytes show an increase in spontaneous calcium transients in vivo in a mouse model of familial AD (FAD) [9] , indicating a hyperactive astrocytic phenotype in AD. However, the signalling pathways underlying this hyperactivity, as well as the possible consequences for cerebrovascular function, have remained unknown. Here we find that astrocytic hyperactivity and calcium waves in a mouse model of FAD are mediated by paracrine purinergic signalling. Inhibition of the release of purinergic messengers through connexin channels as well as purinoreceptor blockade strongly reduce astrocyte hyperactivity. Moreover, we show that this effect is mediated by P2Y receptors but not by P2X receptors. Finally, we show that P2Y1 receptors are strongly expressed by astrocytes around plaques, that an increase of the P2Y1 receptor ligand ADP amplifies hyperactivity and that P2Y1 receptor inhibition normalizes astrocytic network activity. Overall, our data may provide a novel target for the treatment of network dysregulation in AD. Astrocytes are hyperactive near Aβ plaques in APPPS1 mice As a model of FAD, we used mice that co-express the human KM67/671NL mutation in the amyloid precursor protein (APPswe) and human L166P-mutated presenilin 1 (PS1), under the control of the Thy1 promoter (APPPS1) [10] , and their wild-type age-matched littermates. To investigate astrocytic activity in vivo using multiphoton microscopy, we implanted cranial windows over somatosensory cortex in anaesthetized mice. Cells in cortical layers L1–L3 were labelled with the cell-permeable fluorescent calcium indicator Oregon Green BAPTA-1 (OGB-1) AM and the astrocyte marker sulforhodamine 101 (SR101) [11] ( Supplementary Fig. 1a and Supplementary Movie 1 ). Astrocytes were identified by OGB-1 AM and SR101 co-labelling ( Fig. 1a and Supplementary Movie 1 ). In addition, we labelled Aβ plaques with the intravital fluorescent marker methoxy-XO4 [12] ( Fig. 1a and Supplementary Movie 1 ). We chose an anaesthetic regimen that enabled us to use a concentration of isoflurane that has previously shown very little interference with stimulus-evoked calcium responses of cortical astrocytes and cerebrovascular regulation [13] . 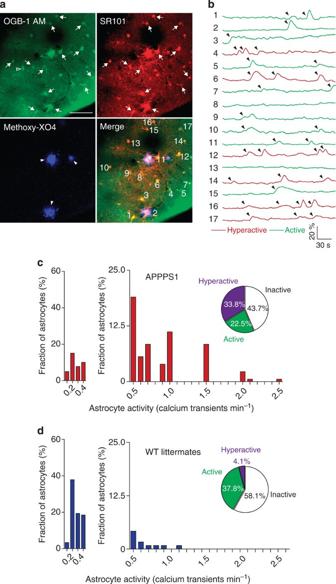Figure 1: Astrocytes are hyperactive in APPPS1 mice. (a,b) Cells were labelled with the green-fluorescent calcium indicator OGB-1 AM and astrocytes were identified by co-labelling with red-fluorescent SR101 (arrows indicate astrocytes identified by double labelling; the open arrowhead illustrates a neuron labelled with OGB-1). Plaques were labelled with the blue-fluorescent plaque marker methoxy-XO4 (arrowheads). In astrocytes positive for both OGB-1 and SR101 (labelled 1–17 ina), spontaneous calcium activity could be detected (arrowheads), ranging from inactive to hyperactive. Inactivity, activity (green traces inb) and hyperactivity (red traces inb) were defined as 0, 0.1–0.4 and >0.4 events per min, respectively. Scale bar, 50 μm. (c,d) Frequency histograms revealed that significantly more astrocytes are hyperactive and less astrocytes are inactive in APPPS1 mice compared with age-matched wild-type littermates (33.8% versus 4.1%;P<0.05,χ2-test; based on 5-min time lapse series fromn=206 astrocytes fromn=9 APPPS1 mice versusn=299 astrocytes fromn=10 wild-type mice and 20-min time-lapse series fromn=69 astrocytes fromn=4 APPPS1 mice versusn=67 astrocytes fromn=3 wild-type mice, respectively). Figure 1: Astrocytes are hyperactive in APPPS1 mice. ( a , b ) Cells were labelled with the green-fluorescent calcium indicator OGB-1 AM and astrocytes were identified by co-labelling with red-fluorescent SR101 (arrows indicate astrocytes identified by double labelling; the open arrowhead illustrates a neuron labelled with OGB-1). Plaques were labelled with the blue-fluorescent plaque marker methoxy-XO4 (arrowheads). In astrocytes positive for both OGB-1 and SR101 (labelled 1–17 in a ), spontaneous calcium activity could be detected (arrowheads), ranging from inactive to hyperactive. Inactivity, activity (green traces in b ) and hyperactivity (red traces in b ) were defined as 0, 0.1–0.4 and >0.4 events per min, respectively. Scale bar, 50 μm. ( c , d ) Frequency histograms revealed that significantly more astrocytes are hyperactive and less astrocytes are inactive in APPPS1 mice compared with age-matched wild-type littermates (33.8% versus 4.1%; P <0.05, χ 2 -test; based on 5-min time lapse series from n =206 astrocytes from n =9 APPPS1 mice versus n =299 astrocytes from n =10 wild-type mice and 20-min time-lapse series from n =69 astrocytes from n =4 APPPS1 mice versus n =67 astrocytes from n =3 wild-type mice, respectively). Full size image Cortical astrocytes were defined as active when their fluorescence increased ≥2 s.d. relative to baseline fluorescence for ≥5 frames (see Methods). In plaque-bearing APPPS1 mice, we found that a large number of astrocytes in cortex were spontaneously active ( Fig. 1a,b and Supplementary Movie 2 ). Based on earlier studies in anaesthetized mice and rats [14] , [15] , [16] , we classified astrocytes as inactive (0 events per min), active (0.1–0.4 events per min) and hyperactive (>0.4 events per min). We found that the fraction of hyperactive astrocytes was significantly larger in transgenic mice compared with age-matched wild-type littermates (33.8% versus 4.1%; Fig. 1c,d ). Moreover, the fraction of inactive astrocytes was significantly smaller in transgenic mice compared with age-matched wild-type littermates (43.7% versus 58.1%; Fig. 1c,d ). Taken together, in APPPS1 mice, similar to an earlier study in another model [9] , there is a relative increase in the population of hyperactive astrocytes on the expense of normal-active and -inactive astrocytes. To investigate whether astrocytic hyperactivity correlates with the vicinity to Aβ plaques, we stained astrocytes in fixed brain sections from transgenic mice for glial fibrillary acid protein (GFAP), a standard marker for reactive astrocytes in cortex. We found that 86% of GFAP-positive reactive astrocytes in the cortex were located within ≤50 μm around plaques ( Fig. 2a ). Therefore, and in accordance with earlier studies [9] , [17] , we dichotomized astrocytes into groups <50 μm and >50 μm away from methoxy-XO4-positive plaques. We found that the relative fraction of hyperactive astrocytes was significantly larger in astrocytes closer to plaques than in those farther away ( Fig. 2b ; 38.2% versus 14.0%), whereas the relative fraction of inactive astrocytes predominated farther away from plaques ( Fig. 2b ; 45.8% versus 26.5%). Regardless of plaque distance, however, the fraction of hyperactive astrocytes always remained higher and that of inactive astrocytes lower, when compared with wild-type littermates. 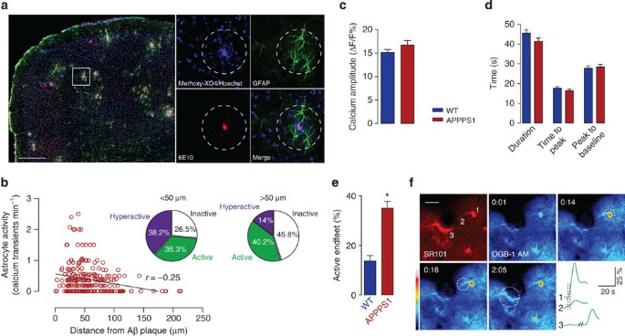Figure 2: Astrocytic hyperactivity correlates with reactive astrogliosis around plaques and involves astrocytic endfeet. (a) Astrocytosis (GFAP staining, green) predominantly occurs <50 μm around plaques (dashed circles). Plaques were double-stained with methoxy-XO4 (blue) and 6E10 antibody (red). Representative image from fixed brain sections fromn=4 analysed mice. Nuclei are stained with Hoechst 33258 (blue). Scale bar, 250 μm. (b) There was a negative correlation between astrocyte activity and distance to plaque (Pearson’sr: −0.25). Overall, significantly more astrocytes were hyperactive and less astrocytes were inactive at a plaque distance <50 μm compared with >50 μm (pie charts; hyperactivity, 38.2% versus 14.0%; inactivity, 26.5% versus 45.8%;n=501 astrocytes fromn=22 mice;P<0.05,χ2-test). (c,d) The relative calcium-evoked fluorescence increase of OGB-1 was similar in APPPS1 mice compared with age-matched wild-type littermates. Similarly, there were no significant differences in the temporal kinetics (total duration, time to peak and peak to baseline) of the calcium signals in both groups (n=175 astrocytes fromn=22 APPPS1 mice versusn=137 astrocytes fromn=18 wild-type littermates;P>0.05, Mann–Whitney test). (e) The fraction of spontaneously active endfeet was higher in APPPS1 mice than in wild-type littermates (35.0±2.7% versus 13.7±2.2%;P<0.05, Mann–Whitney test; the fraction of labelled endfeet was equal in both groups). (f) In astrocytes with active endfeet, we observed calcium elevations that propagated from astrocytic somata into endfeet, as well as calcium elevations that appeared exclusively in endfeet. In this representative time-lapse series, OGB-1 fluorescence (pseudo-coloured) in SR101-positive astrocytes was monitored. In one astrocyte, spontaneous calcium activity occurs first in the soma (1) and subsequently propagates into an endfoot (2). In another astrocyte, calcium elevations appear exclusively in perivascular endfeet (3). Dashed vertical lines indicate onset of signal increase in regions of interest 1–3. Scale bar, 20 μm. Figure 2: Astrocytic hyperactivity correlates with reactive astrogliosis around plaques and involves astrocytic endfeet. ( a ) Astrocytosis (GFAP staining, green) predominantly occurs <50 μm around plaques (dashed circles). Plaques were double-stained with methoxy-XO4 (blue) and 6E10 antibody (red). Representative image from fixed brain sections from n =4 analysed mice. Nuclei are stained with Hoechst 33258 (blue). Scale bar, 250 μm. ( b ) There was a negative correlation between astrocyte activity and distance to plaque (Pearson’s r : −0.25). Overall, significantly more astrocytes were hyperactive and less astrocytes were inactive at a plaque distance <50 μm compared with >50 μm (pie charts; hyperactivity, 38.2% versus 14.0%; inactivity, 26.5% versus 45.8%; n =501 astrocytes from n =22 mice; P <0.05, χ 2 -test). ( c , d ) The relative calcium-evoked fluorescence increase of OGB-1 was similar in APPPS1 mice compared with age-matched wild-type littermates. Similarly, there were no significant differences in the temporal kinetics (total duration, time to peak and peak to baseline) of the calcium signals in both groups ( n =175 astrocytes from n =22 APPPS1 mice versus n =137 astrocytes from n =18 wild-type littermates; P >0.05, Mann–Whitney test). ( e ) The fraction of spontaneously active endfeet was higher in APPPS1 mice than in wild-type littermates (35.0±2.7% versus 13.7±2.2%; P <0.05, Mann–Whitney test; the fraction of labelled endfeet was equal in both groups). ( f ) In astrocytes with active endfeet, we observed calcium elevations that propagated from astrocytic somata into endfeet, as well as calcium elevations that appeared exclusively in endfeet. In this representative time-lapse series, OGB-1 fluorescence (pseudo-coloured) in SR101-positive astrocytes was monitored. In one astrocyte, spontaneous calcium activity occurs first in the soma (1) and subsequently propagates into an endfoot (2). In another astrocyte, calcium elevations appear exclusively in perivascular endfeet (3). Dashed vertical lines indicate onset of signal increase in regions of interest 1–3. Scale bar, 20 μm. Full size image There were no differences in calcium amplitude or duration of calcium transients (total duration, time to peak and peak to baseline) between transgenic and wild-type mice ( Fig. 2c,d ). Recent studies have shown that calcium elevations in astrocytic processes and endfeet may occur independently from somatic calcium changes [18] , [19] . Therefore, we also investigated the involvement of astrocytic processes in spontaneous calcium activity. Only a fraction of endfeet showed discernable OGB-1 AM labelling in APPPS1 (20.9% of 501 OGB-1 labelled astrocytes from n =22 mice) and wild-type mice (15.1% of 496 astrocytes from n =19 mice), probably because multi-cell bolus-loading of calcium indicators mostly labels cell somata [18] . We found that the fraction of spontaneously active endfeet was higher in APPPS1 mice than in wild-type littermates ( Fig. 2e ). We observed calcium elevations that propagated from astrocytic somata into endfeet, as well as calcium elevations that appeared exclusively in endfeet ( Fig. 2f ). The amplitude and duration of calcium elevations in endfeet were comparable in transgenic and wild-type mice (APPPS1 mice, 21.2±1.6% and 26.7±2.8 s, respectively; wild-type littermates, 20.5±2.4% and 31.0±6.3 s, respectively). As we were also interested in the possible relationship between calcium events and changes in arteriolar tone (see below), most data were acquired from layers L1–L2. In experiments in which we recorded from deeper layers, we also identified neuronal somata loaded with OGB-1 ( n =127 neurons in n =7 transgenic mice) that displayed activity levels indicative of hyperactivity ( Supplementary Fig. 1b,c ) as reported [17] , [20] , [21] , [22] . To rule out possible excitatory effects of SR101 (ref. 23 ) in our experiments, we topically applied the calcium indicator rhod-2 AM to specifically label cortical astrocytes [24] in a separate group ( Supplementary Fig. 2a ). We found no difference in astrocyte activity levels in this group compared with mice labelled with OGB-1/SR101 ( Supplementary Fig. 2b ; n =167 astrocytes from n =3 mice). Calcium waves and cerebrovascular changes in APPPS1 mice Calcium waves and propagating calcium events have been observed in some models of neurological diseases [4] , [5] , [25] , including a mouse model of FAD [9] . Therefore, we investigated the occurrence and characteristics of intercellular calcium events, defined as calcium transients that started in one astrocyte, consecutively appeared within ≤3 time frames in immediately adjacent SR101-positive astrocyte somata, and overall involved >2 astrocytes in the imaging plane. We found that intercellular calcium events involving astrocytic somata and processes indeed occurred in APPPS1 mice ( Fig. 3a ). In total, 24 intercellular events occurred in n =13 mice (of a total of 22 mice), travelled for a distance of 120.6±24.1 μm and with a velocity of 9.7±4.8 μm s −1 within the xy imaging plane and had a mean peak calcium amplitude of 27.9±3.4% ( Fig. 3b ). Interestingly, unlike calcium waves initiated by a defined point source such as local application of exogenous ATP [26] , most intercellular calcium events in our experiments, after having first appeared in one astrocyte in the imaging plane, tended to propagate into surrounding astrocytes unidirectionally, and not concentrically. Therefore, to compare these intercellular calcium events to ‘classical’ calcium waves evoked by a defined point source, we triggered calcium waves in vivo by microiontophoretic application of ATP in cortex labelled with OGB-1 AM and SR101 in a separate group. Similar to earlier reports [26] , ATP evoked calcium waves in astrocytes that initiated near the iontophoretic electrode, subsequently propagated into all surrounding astrocytes with a concentric wavefront and spread beyond the field of view ( Fig. 3c ). The velocity of these waves ( Fig. 3d ; 11.2±5.3 μm s −1 , n =6 waves involving n =68 astrocytes from n =2 wild-type mice) was similar to that of spontaneous intercellular events in APPPS1 mice (see above), suggesting that intercellular events in APPPS1 mice may represent ‘true’ calcium waves, and that the unidirectionality of their propagation may be related to a triggering point source outside of the xy imaging plane. 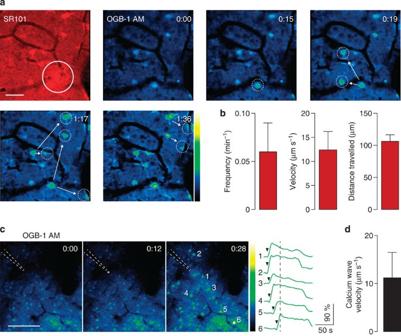Figure 3: Calcium waves in APPPS1 mice. (a) Intercellular calcium events in APPPS1 mice. Astrocytes were identified by SR101 and OGB-1 co-labelling (a nearby plaque is also labelled by SR101 (solid circle)). Time-lapse images in this example show that a calcium signal first appears in an astrocyte soma (dashed circle), and subsequently spreads to neighbouring astrocyte somata and processes (arrows and dashed circles). Scale bar, 30 μm. (b) Frequency, velocity and distance travelled of intercellular calcium events in APPPS1 mice. (c,d) For comparison, we triggered calcium waves by microiontophoresis of ATP in wild-type littermates (n=8 waves involvingn=42 astrocytes inn=2 mice). In this example, astrocytes were labelled with OGB-1 AM and identified by SR101 (not shown). The electrode (indicated by dashed lines in the upper left corner) was filled with ATP and Alexa 594 (red fluorescence, not shown). ATP was delivered in the second image (indicated by asterisk) and triggered a calcium wave with a concentric wavefront. Accordingly, calcium transients at the wavefront were detectable simultaneously in astrocytes at equidistance to the electrode tip (1 and 2; 3 and 4), but successively in astrocytes at different distances to the electrode tip (1–3–5–6; onsets are indicated by black arrowheads on top of corresponding calcium traces; the black vertical dashed line indicates the time point of the right image). Scale bar, 100 μm. The velocity of ATP-evoked calcium waves is given ind. Figure 3: Calcium waves in APPPS1 mice. ( a ) Intercellular calcium events in APPPS1 mice. Astrocytes were identified by SR101 and OGB-1 co-labelling (a nearby plaque is also labelled by SR101 (solid circle)). Time-lapse images in this example show that a calcium signal first appears in an astrocyte soma (dashed circle), and subsequently spreads to neighbouring astrocyte somata and processes (arrows and dashed circles). Scale bar, 30 μm. ( b ) Frequency, velocity and distance travelled of intercellular calcium events in APPPS1 mice. ( c , d ) For comparison, we triggered calcium waves by microiontophoresis of ATP in wild-type littermates ( n =8 waves involving n =42 astrocytes in n =2 mice). In this example, astrocytes were labelled with OGB-1 AM and identified by SR101 (not shown). The electrode (indicated by dashed lines in the upper left corner) was filled with ATP and Alexa 594 (red fluorescence, not shown). ATP was delivered in the second image (indicated by asterisk) and triggered a calcium wave with a concentric wavefront. Accordingly, calcium transients at the wavefront were detectable simultaneously in astrocytes at equidistance to the electrode tip (1 and 2; 3 and 4), but successively in astrocytes at different distances to the electrode tip (1–3–5–6; onsets are indicated by black arrowheads on top of corresponding calcium traces; the black vertical dashed line indicates the time point of the right image). Scale bar, 100 μm. The velocity of ATP-evoked calcium waves is given in d . Full size image As calcium changes in astrocytes have been implicated in the local regulation of CBF [5] , we also investigated whether they are associated with changes of nearby cortical penetrating arterioles. To this end, we simultaneously recorded changes in the diameter of penetrating arterioles (mean diameter at baseline, 12.9±0.6 μm) by injecting dextran-coupled fluorescein isothiocyanate intravenously [27] . Spontaneous blood vessel changes were significantly more frequent in APPPS1 mice than in wild-type littermates (3.1±0.3 versus 1.7±0.2 events per animal; Fig. 4a ). In APPPS1 mice, arteriolar constrictions were more common than dilation (63% versus 37%; Fig. 4b ). Mean diameter change was −12.6±1.6% during vasoconstriction and 14.3±2.1% during vasodilation ( Fig. 4c ). Assuming Hagen–Poiseuille’s law, these diameter changes would result in estimated CBF changes of −39.7±3.9% during vasoconstriction and 79.4±15.2% during vasodilation ( Fig. 4d ). Vasoconstriction and vasodilation were both long-lasting (81.0±7.2 and 84.6±7.2 s, respectively; Fig. 4e ). Interestingly, the duration of vasoconstriction became more severe with age, whereas vasodilations became less pronounced ( Fig. 4f ), indicating that cerebrovascular perturbation increases in parallel with the progression of neuropathological changes, similar to other FAD models [2] . 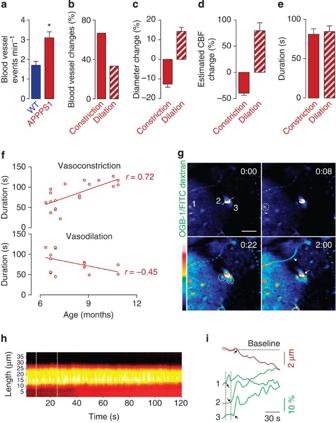Figure 4: Calcium waves and cerebrovascular pathology in APPPS1 mice. (a–e) Cerebrovascular changes in APPPS1 mice. The cross-sectional diameter of penetrating arterioles was studied by injecting dextran-coupled fluorescein isothiocyanate (FITC) intravenously and monitoring changes in diameter in parallel to astrocytic calcium changes. The frequency of CBF changes was significantly higher in APPPS1 mice (a), with arteriolar constriction being common than dilation (b). Assuming Poiseuille’s law, we estimated that diameter changes during vasoconstriction and dilation (c) resulted in strong changes in CBF (d). Vasoconstriction and vasodilation were both long-lasting (e). (f) The duration of vasoconstriction became more severe with age, whereas vasodilations became less pronounced in APPPS1 mice. (g–i) Calcium waves in perivascular astrocytes preceded changes in arteriolar tone in some cases. This example shows a calcium wave associated with vasoconstriction. Astrocytes were labelled with OGB-1 and SR101 (not shown), and blood vessels were labelled with FITC dextran. Time-lapse calcium signals of three astrocytes (labelled 1–3 ing) are displayed (ΔF/F%) ini. Increases of activity in these astrocytes as part of the calcium wave are indicated by dashed circles ing, arrows iniand dashed vertical lines inhandi. Changes in the diameter of the penetrating cortical arteriole were measured by placing a line selection (dashed line ing) through the vessel and creating a cross-sectional image over time by reslicing the line selection (h; see Methods). The inner diameter of the arteriole was identified automatically using a segmentation algorithm and is plotted as the blue horizontal dashed lines inhand as the red trace ini, indicating vasoconstriction. This vasoconstriction is also visible ingas a smaller cross-sectional area of the penetrating arteriole (arrow) and cessation of erythrocyte passage through a nearby capillary (arrowhead). Scale bar, 30 μm. Figure 4: Calcium waves and cerebrovascular pathology in APPPS1 mice. ( a – e ) Cerebrovascular changes in APPPS1 mice. The cross-sectional diameter of penetrating arterioles was studied by injecting dextran-coupled fluorescein isothiocyanate (FITC) intravenously and monitoring changes in diameter in parallel to astrocytic calcium changes. The frequency of CBF changes was significantly higher in APPPS1 mice ( a ), with arteriolar constriction being common than dilation ( b ). Assuming Poiseuille’s law, we estimated that diameter changes during vasoconstriction and dilation ( c ) resulted in strong changes in CBF ( d ). Vasoconstriction and vasodilation were both long-lasting ( e ). ( f ) The duration of vasoconstriction became more severe with age, whereas vasodilations became less pronounced in APPPS1 mice. ( g – i ) Calcium waves in perivascular astrocytes preceded changes in arteriolar tone in some cases. This example shows a calcium wave associated with vasoconstriction. Astrocytes were labelled with OGB-1 and SR101 (not shown), and blood vessels were labelled with FITC dextran. Time-lapse calcium signals of three astrocytes (labelled 1–3 in g ) are displayed (ΔF/F%) in i . Increases of activity in these astrocytes as part of the calcium wave are indicated by dashed circles in g , arrows in i and dashed vertical lines in h and i . Changes in the diameter of the penetrating cortical arteriole were measured by placing a line selection (dashed line in g ) through the vessel and creating a cross-sectional image over time by reslicing the line selection ( h ; see Methods). The inner diameter of the arteriole was identified automatically using a segmentation algorithm and is plotted as the blue horizontal dashed lines in h and as the red trace in i , indicating vasoconstriction. This vasoconstriction is also visible in g as a smaller cross-sectional area of the penetrating arteriole (arrow) and cessation of erythrocyte passage through a nearby capillary (arrowhead). Scale bar, 30 μm. Full size image Although blood vessel changes were common in APPPS1 mice, we detected concomitant spontaneous astrocytic calcium waves in only a fraction of cases ( n =14 events in n =6 mice; vasoconstriction, 8 events, vasodilation, 6 events), whereas no concomitant calcium activity could be observed in the remaining cases of vascular activity. As calcium and vascular activity propagate three dimensionally [28] , whereas our analysis was restricted to the two-dimensional imaging plane, in most cases of accompanying calcium waves we were not able to faithfully determine the temporal relationship between astrocytic calcium elevations and the onset of vessel changes. In six events, however, we recorded calcium waves propagating through perivascular astrocytes, which were followed by local vasodilation or vasoconstriction after a delay of 3–8 s. Examples of calcium waves associated with vasoconstriction and vasodilation, respectively, are presented in Fig. 4g–i and in Supplementary Movie 3 . These data indicate that APPPS1 mice show signs of cerebrovascular pathology, and that although pathways not related to astrocytic calcium activity may be responsible for many aspects of vascular dysregulation in FAD models [2] , [29] , a fraction of vessel changes are associated with simultaneous astrocytic calcium transients. Purinoreceptor signalling underlies astrocytic hyperactivity One way for astrocytes to communicate with their environment is by purinergic signalling, in which paracrine gliotransmitters such as ATP are released through astrocytic connexin hemichannels and evoke glial calcium transients through purinoreceptors [4] , [25] , [30] . In addition, changes in the concentration of purinoreceptor ligands [31] and the expression of purinoreceptors [32] have been described in AD, prompting us to explore the role of purinoreceptors in our model. To this end, we recorded spontaneous calcium activity before and after topical application of modulators of purinergic signalling. We found that pyridoxalphosphate-6-azophenyl-2′,4′-disulfonate (PPADS; 500 μM), a P2 receptor antagonist, strongly reduced the fraction of hyperactive astrocytes to <1% in APPPS1 mice ( Fig. 5a ). Moreover, the connexin channel inhibitor carbenoxolone (100 μM), which inhibits the release of ATP through astrocyte hemichannels [30] , also significantly reduced the fraction of hyperactive astrocytes in APPPS1 mice ( Fig. 5a ). PPADS and carbenoxolone also reduced the frequency of calcium transients in all active astrocytes ( Fig. 5b ). Together, these data indicate that the vast majority of astrocytic hyperactivity in APPPS1 mice is mediated by purinergic signalling. 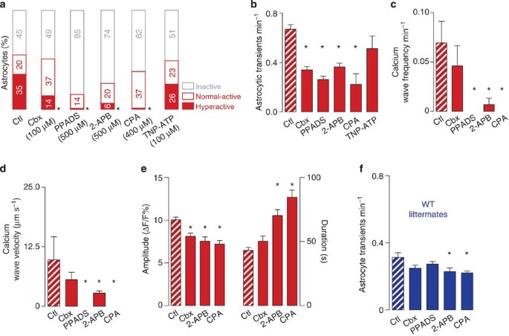Figure 5: Purinergic signalling mediates astrocytic hyperactivity. (a) The connexin channel blocker carbenoxolone (Cbx, 100 μM), the P2 receptor blocker PPADS (500 μM) and the cell-permeable IP3 receptor blocker 2-APB (500 μM) all significantly reduced the frequency of hyperactive astrocytes in APPPS1 mice (Cbx:n=90 astrocytes fromn=4 mice; PPADS:n=228 astrocytes fromn=3 mice; 2-APB:n=134 astrocytes fromn=3 mice; CPA:n=148 astrocytes fromn=4 mice;P<0.05,χ2-test for all groups). In contrast, the P2X receptor blocker TNP-ATP had no effect (n=219 astrocytes fromn=3 mice;P>0.05,χ2-test; 100 μM). Baseline activity was first recorded during topical application of artificial cerebrospinal fluid (Ctl) and again after drug application. (b) Cbx, PPADS, 2-APB and CPA, but not TNP-ATP, also reduced the frequency of astrocyte calcium transients in all active astrocytes (P<0.05, Kruskal–Wallis test followed by Dunn’s multiple comparisons test). (c,d) Inhibition of IP3 receptors (2-APB) significantly reduced the rate and velocity of calcium waves, while inhibition of P2 receptors (PPADS) or depletion of intracellular calcium stores (CPA) completely inhibited calcium waves (P<0.05, Kruskal–Wallis test followed by Dunn’s multiple comparisons test for all). There was a trend for reduction of calcium wave parameters after inhibition of connexin channels with Cbx. (e) Cbx, 2-APB and CPA significantly reduced the amplitude of astrocytic calcium transients. 2-APB and CPA also significantly increased their duration (P<0.05, Kruskal–Wallis test followed by Dunn’s multiple comparisons test for both). (f) Cbx and PPADS had no effect on calcium transients in wild-type littermates, while 2-APB and CPA significantly reduced astrocytic calcium transient frequency in these mice (Kruskal–Wallis test followed by Dunn’s multiple comparisons test; carbenoxolone,n=178 astrocytes fromn=3 mice; PPADS,n=151 astrocytes fromn=3 mice; 2-APB,n=127 astrocytes fromn=3 mice; CPA,n=105 astrocytes fromn=3 mice). Figure 5: Purinergic signalling mediates astrocytic hyperactivity. ( a ) The connexin channel blocker carbenoxolone (Cbx, 100 μM), the P2 receptor blocker PPADS (500 μM) and the cell-permeable IP3 receptor blocker 2-APB (500 μM) all significantly reduced the frequency of hyperactive astrocytes in APPPS1 mice (Cbx: n =90 astrocytes from n =4 mice; PPADS: n =228 astrocytes from n =3 mice; 2-APB: n =134 astrocytes from n =3 mice; CPA: n =148 astrocytes from n =4 mice; P <0.05, χ 2 -test for all groups). In contrast, the P2X receptor blocker TNP-ATP had no effect ( n =219 astrocytes from n =3 mice; P >0.05, χ 2 -test; 100 μM). Baseline activity was first recorded during topical application of artificial cerebrospinal fluid (Ctl) and again after drug application. ( b ) Cbx, PPADS, 2-APB and CPA, but not TNP-ATP, also reduced the frequency of astrocyte calcium transients in all active astrocytes ( P <0.05, Kruskal–Wallis test followed by Dunn’s multiple comparisons test). ( c , d ) Inhibition of IP3 receptors (2-APB) significantly reduced the rate and velocity of calcium waves, while inhibition of P2 receptors (PPADS) or depletion of intracellular calcium stores (CPA) completely inhibited calcium waves ( P <0.05, Kruskal–Wallis test followed by Dunn’s multiple comparisons test for all). There was a trend for reduction of calcium wave parameters after inhibition of connexin channels with Cbx. ( e ) Cbx, 2-APB and CPA significantly reduced the amplitude of astrocytic calcium transients. 2-APB and CPA also significantly increased their duration ( P <0.05, Kruskal–Wallis test followed by Dunn’s multiple comparisons test for both). ( f ) Cbx and PPADS had no effect on calcium transients in wild-type littermates, while 2-APB and CPA significantly reduced astrocytic calcium transient frequency in these mice (Kruskal–Wallis test followed by Dunn’s multiple comparisons test; carbenoxolone, n =178 astrocytes from n =3 mice; PPADS, n =151 astrocytes from n =3 mice; 2-APB, n =127 astrocytes from n =3 mice; CPA, n =105 astrocytes from n =3 mice). Full size image As PPADS is an antagonist of many different P2X and P2Y receptors, we subsequently aimed to investigate which purinoreceptor subtype is responsible for astroglial hyperactivity. We found that TNP-ATP (100 μM), a blocker of P2X receptors [33] , had no effect on the fraction of hyperactive astrocytes or the frequency of calcium transients in all active astrocytes ( Fig. 5a,b ). As astrocytes express different P2Y receptors [34] and no broad-spectrum P2Y receptor blockers exist to our knowledge, we first explored their possible contribution to astrocytic hyperactivity by applying 2-Aminoethoxydiphenyl borate (2-APB; 500 μM), a cell-permeable blocker of inositol 1,4,5-trisphosphate (IP3) receptors [35] , which mediate P2Y receptor-evoked calcium release from the endoplasmic reticulum [34] . 2-APB significantly reduced the fraction of hyperactive astrocytes ( Fig. 5a ) and the frequency of calcium transients in all active astrocytes ( Fig. 5b ). As 2-APB also has effects on targets other than IP3 receptors [36] , we performed additional experiments using cyclopiazonic acid (CPA; 400 μM), a specific endoplasmic reticulum calcium ATPase inhibitor [37] , to test whether astrocytic transients depended on calcium release from intracellular stores. We found that CPA significantly reduced the fraction of hyperactive astrocytes to 1% in APPPS1 mice ( Fig. 5a ) and significantly reduced the frequency of calcium transients in all active astrocytes ( Fig. 5b ). In addition, PPADS and CPA completely inhibited, 2-APB significantly reduced and carbenoxolone showed a trend towards a reduction of the frequency and velocity of calcium waves ( Fig. 5c,d ). Moreover, 2-APB, CPA and carbenoxolone slightly, but significantly, reduced the amplitude of astrocytic calcium transients ( Fig. 5e ). 2-APB and CPA, but not carbenoxolone, also increased their duration ( Fig. 5e ) similar to earlier reports [38] . In contrast to APPPS1 mice, carbenoxolone and PPADS had no effect on the frequency of astrocytic calcium transients in age-matched wild-type littermates, similar to what has been reported in other studies for anaesthetized and awake animals, as well as acute brain slices [15] , [39] , [40] . 2-APB and CPA reduced astrocytic calcium transient frequency in wild-type mice as well ( Fig. 5f ). These data indicate that release of ATP through connexin channels and P2Y receptor signalling contribute to astrocytic hyperactivity and cell-to-cell propagation of astrocyte activity in APPPS1 mice, but not in wild-type mice. The age of animals and their cortical plaque load were comparable between all groups ( Supplementary Table 1 ). P2Y1 receptor blockade normalizes astrocytic hyperactivity Next, we aimed to pinpoint which P2Y receptor subtype is responsible for astrocytic hyperactivity. Astrocytes have been found to express P2Y1, P2Y2 and P2Y4 in the cortex in situ [34] . P2Y2 receptor expression is reduced [41] , while P2Y1 receptor expression is enhanced in AD [42] , prompting us to focus on the role of P2Y1 receptors in astrocytic hyperactivity. P2Y1 receptors are relatively insensitive to ATP, but are strongly activated by ADP [43] . We therefore reasoned that if P2Y1 receptors mediate astrocytic hyperactivity in our model, an increase in the concentration of ADP in the tissue should result in increased astrocyte signalling. Therefore, we topically applied a grade of apyrase ectonucleotidase (300 U ml −1 ) that preferentially contains ATPase activity, but much lesser ADPase activity and very little AMPase activity, to increase the ADP concentration by accelerating ATP hydrolysis but minimizing ADP degradation [43] , [44] . We found that this treatment resulted in strongly enhanced overall astrocytic activity in APPPS1 mice ( Fig. 6a ) and a significantly higher fraction of hyperactive astrocytes compared with the fractions before apyrase application ( Fig. 6b ). Moreover, we found that apyrase treatment resulted in a significant increase in the rate of astrocytic calcium waves ( Fig. 6c ). Calcium wave velocities and distances travelled did not change significantly after apyrase application ( Fig. 6d,e ). 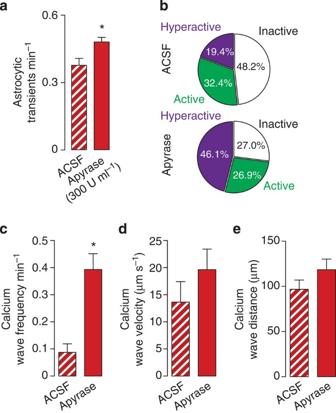Figure 6: Increasing ADP availability by apyrase application amplifies astrocytic hyperactivity and calcium waves. (a) Augmenting the hydrolysis of ATP to ADP, while minimizing ADP degradation, using the ectonuleotidase apyrase significantly increased the frequency of astrocytic transients in all active astrocytes (P<0.05, Mann–Whitney test;n=126 astrocytes fromn=3 mice). (b) Apyrase significantly increased the fraction of hyperactive astrocytes and decreased the fraction of inactive astrocytes in APPPS1 mice (P<0.05,χ2-test). (c) Apyrase significantly increase the frequency of astrocytic calcium waves in APPPS1 mice (P<0.05, Mann–Whitney test). (d,e) There was a nonsignificant trend towards a higher velocity of calcium waves after apyrase treatment. No significant difference was observed in the maximal distance calcium waves propagated within the imaging plane (P>0.05, Mann–Whitney test for both). Figure 6: Increasing ADP availability by apyrase application amplifies astrocytic hyperactivity and calcium waves. ( a ) Augmenting the hydrolysis of ATP to ADP, while minimizing ADP degradation, using the ectonuleotidase apyrase significantly increased the frequency of astrocytic transients in all active astrocytes ( P <0.05, Mann–Whitney test; n =126 astrocytes from n =3 mice). ( b ) Apyrase significantly increased the fraction of hyperactive astrocytes and decreased the fraction of inactive astrocytes in APPPS1 mice ( P <0.05, χ 2 -test). ( c ) Apyrase significantly increase the frequency of astrocytic calcium waves in APPPS1 mice ( P <0.05, Mann–Whitney test). ( d , e ) There was a nonsignificant trend towards a higher velocity of calcium waves after apyrase treatment. No significant difference was observed in the maximal distance calcium waves propagated within the imaging plane ( P >0.05, Mann–Whitney test for both). Full size image Next, based on immunohistochemistry of fixed brain sections, we found that P2Y1 receptors are predominantly expressed by reactive astrocytes around Aβ plaques in APPPS1 mice ( Fig. 7a ), similar to what has been reported for reactive astrocytes in other disease models [45] . These data indicate that the areas in which astrocyte activity is highest and P2Y1 receptor expression is strongest show a high spatial overlap. 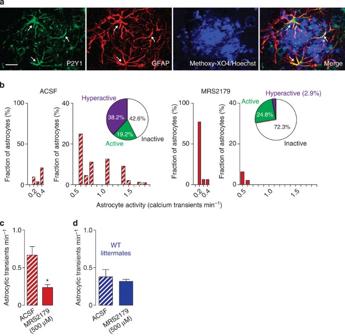Figure 7: P2Y1 receptor inhibition normalizes astrocytic hyperactivity. (a) P2Y1 receptors are predominantly expressed by reactive astrocytes (stained with GFAP antibody; arrows indicate co-expression) around Aβ plaques (stained with methoxy-XO4), indicating a strong spatial overlap of P2Y1 receptor expression and the area where astrocytic hyperactivity is highest. Scale bar, 20 μm. (b) Frequency histogram revealed that the fraction of hyperactive astrocytes was significantly reduced after P2Y1 inhibition in APPPS1 mice (P<0.05,χ2-test), while the fraction of active astrocytes remained unchanged. (c) The P2Y1 receptor blocker MRS2179 significantly reduced the frequency of astrocyte activity in all active astrocytes (n=123 astrocytes fromn=4 mice; 0.67±0.11 versus 0.22±0.20 transients per min;P<0.05, Mann–Whitney test; 500 μM). Baseline activity was recorded during topical application of ACSF and again after drug application. (d) In contrast, MRS2179 had no influence on the frequency of spontaneous astrocyte activity in wild-type littermates (n=111 astrocytes fromn=3 mice;P>0.05, Mann–Whitney test). Figure 7: P2Y1 receptor inhibition normalizes astrocytic hyperactivity. ( a ) P2Y1 receptors are predominantly expressed by reactive astrocytes (stained with GFAP antibody; arrows indicate co-expression) around Aβ plaques (stained with methoxy-XO4), indicating a strong spatial overlap of P2Y1 receptor expression and the area where astrocytic hyperactivity is highest. Scale bar, 20 μm. ( b ) Frequency histogram revealed that the fraction of hyperactive astrocytes was significantly reduced after P2Y1 inhibition in APPPS1 mice ( P <0.05, χ 2 -test), while the fraction of active astrocytes remained unchanged. ( c ) The P2Y1 receptor blocker MRS2179 significantly reduced the frequency of astrocyte activity in all active astrocytes ( n =123 astrocytes from n =4 mice; 0.67±0.11 versus 0.22±0.20 transients per min; P <0.05, Mann–Whitney test; 500 μM). Baseline activity was recorded during topical application of ACSF and again after drug application. ( d ) In contrast, MRS2179 had no influence on the frequency of spontaneous astrocyte activity in wild-type littermates ( n =111 astrocytes from n =3 mice; P >0.05, Mann–Whitney test). Full size image Finally, we tested the P2Y1 receptor-specific inhibitor MRS2179 (500 μM) [46] . Frequency distribution histograms of astrocytic transients before and after application of MRS2179 revealed that the fraction of hyperactive astrocytes was strongly reduced, while the fraction of normal-active astrocytes remained unchanged ( Fig. 7b ). Moreover, the drug significantly reduced the frequency of astrocytic transients in all active astrocytes ( Fig. 7c ). Interestingly, MRS2179 had no significant effect on astrocytic activity in wild-type littermates ( Fig. 7d ). These data indicate that P2Y1 receptor blockade normalizes astrocytic hyperactivity in this model of FAD. Astrocytic and neuronal activity are independent The population of hyperactive neurons around plaques is increased in the cortex and hippocampus in mouse models of FAD [17] , [20] , [21] . As astrocytes respond to neuronal activity [4] , we also tested whether hyperactivity of astrocytes is influenced by neuronal hyperactivity. First, we blocked neuronal transmission by topically applying the voltage-gated sodium channel blocker tetrodotoxin (TTX; 1 μM). To confirm the efficacy of TTX at this concentration and at the cortical depth at which most data were acquired, we recorded the electrocorticogram with a glass electrode inserted into the cortex at the approximate imaging depth in a separate group ( n =3 mice). TTX treatment significantly decreased electrocorticogram amplitude by 77% ( Fig. 8a,b ), indicating sufficient blockade of neuronal activity. However, in APPPS1 mice as well as in wild-type littermates, there was no change in the amplitude and duration of astrocytic calcium signals ( Fig. 8c ). Moreover, the relative fractions of inactive, normally active and hyperactive astrocytes in APPPS1 and wild-type mice remained similar before and after TTX treatment ( Fig. 8d ), and there were no significant differences in the rate or velocity of calcium waves ( Fig. 8e,f ). In addition, we also confirmed that activity of neuronal somata, recorded from L3 neurons labelled with OGB-1 in a subset of recordings, was absent after TTX treatment ( Fig. 8g ). 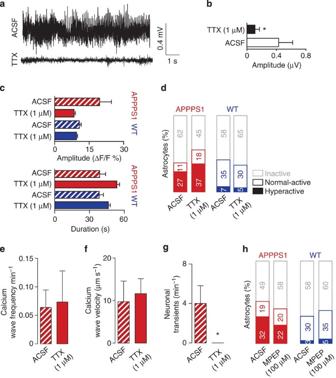Figure 8: Neuronal activity or neuron-to-astrocyte signalling do not mediate astrocytic hyperactivity in APPPS1 mice. (a,b) We blocked neuronal transmission by topically applying the voltage-gated sodium channel blocker TTX (1 μM). Efficacy was confirmed by recording the electrocorticogram before and after TTX. TTX treatment significantly decreased electrocorticogram (ECoG) amplitude by 77% (n=30 15-s epochs before and after TTX application fromn=3 mice;P<0.05, Wilcoxon matched-pairs signed-rank test). (c) In APPPS1 mice as well as in wild-type littermates, there was no change in the amplitude and duration of calcium signals before and after application of TTX (P>0.05, Kruskal–Wallis test followed by Dunn’s multiple comparisons test;n=93 astrocytes fromn=3 APPPS1 mice;n=173 astrocytes fromn=3 wild-type mice). (d) TTX had no effect on the relative fractions of inactive, active or hyperactive astrocytes in APPPS1 mice and wild-type littermates. (P>0.05,χ2-test). (e,f) The rate and velocity of calcium waves remained unchanged after application of TTX in APPPS1 mice (P>0.05, Mann–Whitney test). (g) Neuronal calcium changes, recorded from somata in layer L3, were blocked by TTX (n=17 neurons fromn=2 APPPS1 mice;P<0.05, Mann–Whitney test). (h) No effect on the relative fractions of inactive, active or hyperactive astrocytes were seen in APPPS1 mice and wild-type littermates when we blocked neuron-to-astrocyte signalling with the metabotropic glutamate receptor MPEP (P>0.05,χ2-test; APPPS1,n=122 astrocytes fromn=3 mice; wild-type,n=47 astrocytes fromn=2 mice; 100 μM). Figure 8: Neuronal activity or neuron-to-astrocyte signalling do not mediate astrocytic hyperactivity in APPPS1 mice. ( a , b ) We blocked neuronal transmission by topically applying the voltage-gated sodium channel blocker TTX (1 μM). Efficacy was confirmed by recording the electrocorticogram before and after TTX. TTX treatment significantly decreased electrocorticogram (ECoG) amplitude by 77% ( n =30 15-s epochs before and after TTX application from n =3 mice; P <0.05, Wilcoxon matched-pairs signed-rank test). ( c ) In APPPS1 mice as well as in wild-type littermates, there was no change in the amplitude and duration of calcium signals before and after application of TTX ( P >0.05, Kruskal–Wallis test followed by Dunn’s multiple comparisons test; n =93 astrocytes from n =3 APPPS1 mice; n =173 astrocytes from n =3 wild-type mice). ( d ) TTX had no effect on the relative fractions of inactive, active or hyperactive astrocytes in APPPS1 mice and wild-type littermates. ( P >0.05, χ 2 -test). ( e , f ) The rate and velocity of calcium waves remained unchanged after application of TTX in APPPS1 mice ( P >0.05, Mann–Whitney test). ( g ) Neuronal calcium changes, recorded from somata in layer L3, were blocked by TTX ( n =17 neurons from n =2 APPPS1 mice; P <0.05, Mann–Whitney test). ( h ) No effect on the relative fractions of inactive, active or hyperactive astrocytes were seen in APPPS1 mice and wild-type littermates when we blocked neuron-to-astrocyte signalling with the metabotropic glutamate receptor MPEP ( P >0.05, χ 2 -test; APPPS1, n =122 astrocytes from n =3 mice; wild-type, n =47 astrocytes from n =2 mice; 100 μM). Full size image Next, we investigated the role of neuron-to-astrocyte signalling through metabotropic glutamate receptor 5 (mGluR5), which has been implicated as a target for neuron-derived glutamate on astrocytes [5] . However, topical application of the mGluR5 inhibitor 2-methyl-6-(phenylethynyl)pyridine (MPEP; 100 μM) had no effect on the fraction of inactive, active and hyperactive astrocytes, respectively, in APPPS1 mice and in wild-type littermates ( Fig. 8h ). Together, these results indicate that neuronal transmission, similar to an earlier report [9] , as well as neuron-to-astrocyte signalling do not contribute to astrocytic hyperactivity in APPPS1 mice. In this study, we investigated spontaneous network activity of astrocytes in a mouse model of FAD and found that astroglial hyperactivity was largely mediated by purinergic activity and, in particular, by P2Y1 receptors. A central element of the pathogenesis of AD is the progressive accumulation of Aβ species, ultimately resulting in the formation of Aβ plaques [1] . The paths by which Aβ leads to neurodegeneration are probably multifactorial and include induction of hyperphosphorylated tau aggregation [1] , inflammation [47] , as well as cerebrovascular effects [2] , [29] . In addition, it has become increasingly apparent in recent years that the accumulation of Aβ induces severe and widespread network dysfunction [3] . Thus, epileptiform activity and increased proportions of abnormally hypoactive and hyperactive neurons were observed in animal models [3] , [17] , [20] , [21] . Moreover, network dysfunction also exists in AD patients [3] and even in non-demented but amyloid-positive individuals [48] , suggesting an early and perhaps causal role of network imbalance for cognitive decline. Astrocytes are an integral part of synaptic transmission, regulate brain energetics and mediate cerebrovascular function, and therefore are critical for the establishment and maintenance of neuronal health [4] , [5] . Reactive astrogliosis is a central hallmark of essentially every type of acute or chronic neuronal injury, including AD [7] , but the functional consequences of this transition from the normal to the reactive phenotype have remained largely unknown. Astrocytes in the healthy brain are organized into dynamic networks [25] . Importantly, the expression of molecular components that govern these networks, such as connexin channels, is altered under pathological conditions [25] , indicating that similar to neuronal ensembles, AD is also associated with a perturbation of astrocytic network activity triggered by reactive astrogliosis. Indeed, in vivo evidence of astrocytic network disruption has been observed in previous studies [9] , [22] , [49] , [50] , but the signalling pathways underlying these changes have remained unknown. Here we found that pathological astroglial network activity—intercellular calcium waves as well as single-cell astrocyte hyperactivity—is driven by purinergic signalling. This is in contrast to spontaneous astrocyte activity in anaesthetized or awake wild-type animals and brain slices, which is insensitive to purinoreceptor inhibition, as shown in this and other studies [15] , [39] , [40] . Moreover, we showed that P2Y receptors, and P2Y1 receptors in particular, are responsible for the majority of astroglial hyperactivity. First, we showed that PPADS, a broad-spectrum (but non-universal) purinergic antagonist of P2X and P2Y receptors, strongly attenuated hyperactivity. Second, P2X receptor blockade had no effect, while inhibition of intracellular IP3 receptors or depletion of intracellular calcium stores reduced astroglial hyperactivity, compatible with a role for metabotropic signalling through P2Y receptors. The fact that calcium activity was significantly reduced, but not blocked completely, may be related to differences in the penetration depth or distribution of drugs in vivo , or to a possible involvement of other pathways. Third, increasing the relative concentration of ADP by stimulating the hydrolysis of ATP to ADP with an apyrase that possesses a high ATPase/ADPase activity ratio increased astrocytic hyperactivity and calcium waves, suggesting a predominant role of ADP-sensitive P2Y receptors such as the P2Y1 receptor. Fourth, we found that the areas with highest astroglial hyperactivity were spatially correlated with the strongest levels of astrogliosis, and that P2Y1 receptor expression was also highest in reactive astrocytes around plaques, indicating that astrocytic network disruption was driven by P2Y1 receptor activity in reactive astrocytes. Finally, we showed that P2Y1 receptor blockade completely normalized astroglial network dysfunction. The consequences of P2Y1 receptor-induced hyperactivity, or its normalization by P2Y1 antagonists, remain to be determined. However, it is interesting to note that many functions of P2Y1 receptors—for example, learning and memory [51] , inflammatory responses [52] and synaptic transmission [53] —are strongly perturbed in AD, indicating that P2Y1 receptor modulation may not only normalize astroglial networks, but may also help to ameliorate inflammation and cognitive decline. Interestingly, we found that blocking the release of ATP through connexin hemichannels also attenuated hyperactivity. Earlier studies have shown that connexin hemichannels, which are the main constituents of ATP release [51] , are upregulated via Aβ-dependent mechanisms in astrocytes particularly around Aβ plaques in FAD mouse models [54] , that is, in the areas where astroglial hyperactivity was highest in our study. Moreover, studies in AD patients have demonstrated increased levels of ATP in plaque-bearing brain regions compared with age-matched non-demented control individuals [31] , [55] . Overall, these data suggest that in addition to hyperactivity mediated by P2Y1 receptor upregulation, increased release of ATP through astroglial connexin hemichannels also contributes to astroglial network dysfunction. Of note, earlier studies have reported that exposure of cultured rat astrocytes to Aβ led to astrocytic calcium dysregulation through different mechanisms than the ones identified in our study. Calcium changes evoked by mGluR5 agonists were potentiated by pre-exposure to Aβ in astroglial cultures [56] , [57] , whereas we did not observe a dependence of astrocytic hyperactivity on neuronal transmission or mGluR5 activity. Besides elementary differences between cultured and in vivo astrocytes [58] , it should be noted that the aforementioned studies were performed on cultured astrocytes derived from neonatal animals, in which mGluR5 expression appears to be much higher than in older animals [59] . Moreover, these studies also revealed striking differences between astroglial cultures derived from hippocampi compared with entorhinal cortex [56] , whereas we studied neocortical astrocytes, indicating substantial regional heterogeneities, similar to what has been reported for neuronal hyperactivity in cortex versus hippocampus [21] . In other studies using cultured astrocytes, it was reported that astroglial calcium elevations evoked by high concentrations of Aβ were triggered by oxidative stress and activation of NADPH oxidase [60] . Interestingly, in addition to the canonical metabotropic pathway via IP3 receptors, P2Y1 receptor activation can also lead to activation of NADPH oxidase and generation of free radicals [61] , indicating that P2Y1 receptors may evoke calcium imbalance through multiple pathways. Moreover, P2Y1 receptor inhibition has also been shown to ameliorate tissue damage in animal models of stroke and traumatic brain injury [45] , [62] , but whether astroglial network dysfunction contributes to these diseases remains to be determined. Although the incident laser power has been shown to influence astrocyte activity levels [63] , it is unlikely that this had a significant influence on our data, as we kept the laser power within a range that has been shown to minimize laser-induced artefacts [63] and as spontaneous activity levels of astrocytes in our study was comparable to that in other reports [9] , [15] , [63] . Interestingly, however, lower activity levels were found in another study [49] , indicating that the separation into active and hyperactive astrocytes and neurons used here and in earlier studies [9] , [17] , [22] is relatively arbitrary and that shifts in frequency spectrums between disease models and their controls might better describe the data. One caveat is that our study, as well as all other in vivo studies on astrocytes in FAD models to date, was performed in mice under anaesthesia, which has been shown to influence astrocyte activity levels [39] . Although we used an isoflurane concentration that had previously shown very little influence on stimulus-induced astrocytic calcium changes [13] and astrocyte activity levels in our experiments were comparable to those of awake mice [39] , we cannot rule out an influence of anaesthesia on astrocyte activity. Importantly, however, the main results of our study—significant differences in astrocytic activity and signalling pathways in wild-type and transgenic animals—cannot be attributed to anaesthesia. Nevertheless, it will be important to study neuronal and glial networks in awake animals in FAD models in the future. Another finding in our study was that APPPS1 mice display propagating intercellular calcium events, which—based on their temporal kinetics—probably represent ‘classical’ astroglial calcium waves. Moreover, we detected long-lasting spontaneous vasoconstrictions, which became more severe with age, and vasodilations that became less severe, indicating cerebrovascular deterioration as a consequence of AD-related pathology in this line. CBF perturbations have also been observed in other FAD models [64] , but it is interesting to note that amyloid angiopathy is scarce in APPPS1 mice compared with other models [10] , suggesting that some CBF changes are triggered by mechanisms unrelated to perivascular amyloid deposits. Astrocytic processes completely cover most blood vessels in the brain and astroglial calcium elevations have been implicated in local cerebrovascular regulation [5] . Interestingly, however, we found here that spontaneous CBF changes were preceded by calcium waves involving perivascular astrocytes in only a fraction of cases. These data indicate that other mechanisms, such as vascular oxidative stress, TGF-β signalling or blood–brain barrier alterations [2] , [29] , [64] , prevail in the dysregulation of CBF in AD. However, as changes observed in intracortical vessels can also result from CBF alterations in distant upstream vessels [5] , and as calcium waves and CBF changes both propagate three dimensionally in the brain [28] , the proportion of spontaneous CBF changes accompanied by astrocytic calcium waves is probably higher. Another interesting point is that astrocytic calcium elevations in wild-type animals are associated with vasodilation [5] , whereas in the present study they were associated with vasoconstriction and vasodilation in APPPS1 mice. Future studies will be necessary to determine whether these differences are related to the underlying pathological phenotype, or if neuronal activation, which was not involved in the calcium transients studied here, but triggers vasoactive astrocytic calcium changes under physiological conditions [5] , may facilitate dilatory rather than constrictive vessel responses. Finally, it should also be noted that bulk-loading of pharmacological calcium indicators mostly enables the detection of somatic astrocytic calcium signals, but is relatively insensitive to calcium changes in distant astrocytic compartments such as the perivascular space [18] , suggesting that the use of novel membrane-anchored genetic indicators [19] may help to better understand the role of glio-vascular signalling in AD models in future studies. In summary, we have shown that astroglial network dysfunction is mediated by purinergic signalling in reactive astrocytes, and that modulation of P2Y1 receptor activity or nucleotide release through hemichannels may represent novel targets to ameliorate network dysfunction in AD. Mouse line and cranial window preparation All experiments were performed according to animal care guidelines and approved by local animal welfare committees. We used 5- to 9-month-old mice of both sexes that co-express the human KM67/671NL mutation in the amyloid precursor protein (APPswe) and human L166P-mutated PS1 under the control of the Thy1 promoter on a C57BL/6J background [10] (APPPS1-21; provided by Dr M. Jucker, Tübingen) and their wild-type age-matched and sex-matched littermates. Animals were housed in groups on a 12-h light/dark cycle with food and water available ad libitum . During surgery, animals were anaesthetized with isoflurane (1.5% v/v) and kept on a heating plate (37 °C). After fixation in a stereotaxic frame, the scalp was removed and a 3 × 3 mm craniotomy was created over the left somatosensory cortex using a dental drill as previously described [27] . The dura was removed when pharmacological agents were topically applied. Agarose (2%) was placed on top of the cortex for stabilization and windows were closed with a cover glass (diameter 3 mm) and sealed with silicone elastomer (Kwik-Sil, World Precision Instruments). We performed immunohistochemical analyses of the cranial window area in a subset of animals ( n =3) and found no signs of tissue damage ( Supplementary Fig. 3 ). In vivo two-photon microscopy To visualize Aβ plaques, mice received an intraperitonal injection of Methoxy-XO4 (2–5 mg kg −1 ; solubilized in PBS with 4% Cremophor EL; provided by Dr W. Klunk, University of Pittsburgh) 24 h before cranial window preparation [12] . To visualize calcium activity in cortical astrocytes, the calcium-sensitive dye OGB-1 AM (Invitrogen; solubilized in 20% Pluronic and 80% dimethylsulfoxide and diluted to 1 mM with artificial cerebrospinal fluid, ACSF) and the astrocyte-specific marker SR101 (100 μM) were co-injected into the cortex at a depth of 100–200 μm using glass micropipettes (4–10 μm tip diameter; World Precision Instruments) connected to a pneumatic injector (1 bar, 60–90 s; PDES, NPI Electronic). In some experiments, rhod-2 AM (2 mM) was topically applied to the cortex for 45 min, followed by a brief irrigation with ACSF. To visualize the vasculature, 70 kDa dextran-coupled fluorescein isothiocyanate (5% in ACSF, 100 μl; Sigma) was injected intravenously. During imaging, mice were anaesthetized with a combination of isoflurane (0.4% v/v in 5% O 2 ) and ketamine (50 mg ml −1 ; 10 μl bolus followed by 1.5 μl min −1 , administered through an intraperitoneal catheter connected to a syringe pump), and kept on a homeothermic heating pad. The level of anaesthesia was assessed by testing motor responses to tail pinch. One set of transgenic and wild-type mice was imaged using an upright two-photon microscope (LaVision Trim ScopeII) with a × 20 objective (1.0 numerical aperture, Zeiss) and three non-descanned detectors (420–500, 525–580 and >585 nm) at 253 × 253 pixels (0.5 μm per pixel). Fluorophores were excited at 800 nm using a Ti:Sapphire laser (Chameleon Ultra II, pumped by an 18 W laser, Coherent) with a 140 fs pulse width, 80 MHz repetition rate and an average pixel dwell time of 1.9 μs. A smaller set of transgenic and wild-type mice were imaged using a TCS SP2 upright two-photon microscope (Leica) with a × 20 objective (0.5 numerical aperture, Leica) and two non-descanned detectors (500–550 and 570–650 nm) at 256 × 256 pixels. Fluorophores were excited at 800 nm using a Ti:Sapphire laser (Tsunami, pumped by a 5 W laser, Spectra Physics) with 80 fs pulse width, 82 MHz repetition rate and an average pixel dwell time of 4.9 μs. The intensity point spread functions of both microscopes were 435±49 and 946±63 nm, respectively. Laser power below the objective was kept between 20 and 40 mW to minimize laser-induced artefacts and phototoxicity [63] . Z stacks of the imaging region were taken and XY time-lapse series of spontaneous calcium activity, blood vessels and plaques were subsequently recorded for 2–5 min at 1–3 Hz, or for 20 min at 1 Hz, at a depth of 100–200 μm beneath the surface. Data analysis Mice were excluded if visual damage or bleeding occurred. Otherwise, no samples were excluded from the analysis. Data analysis was performed blinded for pharmacological intervention or genotype unless plaque characteristics were part of the analysis. The coefficient of variation as an estimate of interindividual variability was similar across all groups ( Supplementary Table 1 ). Sample sizes were similar to those used in previous similar studies [9] , [39] , [50] . Time-lapse series were imported into ImageJ 1.48 (W. Rasband, NIH), smoothed using a Gaussian filter and co-registered to an 8-bit grey level image stack using the TurboReg/Stackreg plugins (P. Thévenaz, Lausanne). Only astrocytes positive for both OGB-1 and SR101 were analysed. Neurons were identified by their morphology and the absence of SR101. Neuronal soma as well as astrocytic soma and endfeet regions of interest were set manually using ImageJ, mean fluorescence over time was determined for each regions of interest and then converted to Δ F / F . Cells were defined as active when fluorescence increased ≥2 s.d. relative to baseline fluorescence for a duration of ≥5 frames (astrocytes) or ≥3 frames (neurons). Each time-lapse series that met this criterion was plotted together with the respective video file for visual inspection and verification. Intercellular calcium events were defined as calcium transients (defined as above) that started in one astrocyte, consecutively appeared within ≤3 time frames in immediately adjacent SR101-positive astrocyte somata and, overall, involved >2 astrocytes in the xy imaging plane. Astrocytes that showed a coincidental calcium elevation, but were not located directly adjacent to another active astrocyte, were excluded from this analysis. Ellipses were fit to the maximum extent between active somata to determine the spatial range using ImageJ. Velocity was calculated by dividing the maximal distance between somata by the time lag between respective peaks of calcium transients. For all calcium signals, amplitude, time to peak, peak to baseline and overall duration of the response were determined. Cell-to-cell and cell-to-plaque distances were measured from midpoint to midpoint and cell-to-vessel distance from midpoint to adjacent vessel wall using ImageJ. Vessel diameters were measured semi-automatically by a custom-written plugin for ImageJ (E. Kadas, Berlin). Briefly, a line selection was manually placed through the vessel of interest along its longest axis using ImageJ. Cross-sectional images over time were obtained by creating a resliced image of the line selection and smoothed using a Gaussian filter. The inner diameter of the vessel was identified automatically using a segmentation algorithm, and duration as well as change of diameter relative to baseline were measured. Relative changes in CBF were estimated using Hagen-Poiseuille’s law (assuming constant pressure drop, viscosity and vessel length during the imaging period). Data were obtained in two separate laboratories, analysed separately and subsequently pooled. Plaque load was quantified by determining the area covered by methoxy-XO4 signal relative to total cortical area in binarized images using ImageJ. For analysis of the relative fractions of hyperactive/active/inactive astrocytes, only time-lapse series of 5 and 20 min duration were analysed. Neurons were defined as hypoactive, active or hyperactive based on criteria from earlier studies [17] (hypoactive, 0–0.25 events per min; active, 0.26–4 events per min; hyperactive, >4 events per min). Immunohistochemistry Mice were killed with an overdose of ketamine. The brain was quickly dissected and one hemisphere was fixed in 4% paraformaldehyde for 1 day for immunohistochemistry. Paraformaldehyde-fixed hemispheres were post fixed in sucrose solutions (15 and 25%) containing 0.1% sodium azide for 1 day each, and embedded in cryo-protectant. Coronal sections (20μm) were obtained using a cryostat (Leica) and mounted onto slides. After blocking with 5% normal goat serum (Vector Labs) and 0.25% Triton-X100 (Sigma) in PBS for 1 h, sections were incubated with mouse anti-6E10 (1:1,000; SIG-39300, Covance), rabbit anti-GFAP (1:1,000; Z0334, Dako), rat anti-GFAP (1:1,000; 13-0300, Invitrogen), rabbit anti-P2Y1R (1:200; APR-009, Alomone), rabbit anti-Iba1 (1:500; 019-19741, Wako), or mouse anti-NeuN (1:200; MAB377, Millipore) antibodies, respectively, in blocking solution over night at 4 °C. Stainings were visualized with secondary antibodies from goat conjugated with Cy2, Cy3 and Cy5, respectively (1:1,000; Dianova; 2 h at room temperature). Nuclei were stained with Hoechst 33258 (1:1,000; Invitrogen) and sections were mounted in DePeX (Serva). Confocal images were acquired using a confocal laser scanning microscope (LSM 700; Zeiss) and analysed using ImageJ. NeuN-positive neurons and area covered by GFAP-positive astrocytes and Iba1-positive microglia were determined after binarization using ImageJ. Electrophysiology Mice were anaesthetized with isoflurane, kept on a heating plate and fixed in a stereotaxic frame as described above. A cranial window was prepared as described above. A glass microelectrode (World Precision Instruments; tip diameter, 2–4 μm) containing ACSF was inserted 150–200 μm below the pial surface and a reference electrode was placed subcutaneously at the neck. The electrocorticogram signal was amplified 1,000-fold, bandpass-filtered at 3–100 Hz and digitized at 10 kHz (micro1401, CED). Recordings were analysed offline using Spike2 (CED). Pharmacology All drugs and fluorescent indicators were solubilized in ACSF (in mM: 132 NaCl, 3 KCl, 0.6 MgCl 2 , 1.5 CaCl 2 , 24.6 NaHCO 3 , 3.7 glucose, 6.7 urea). MPEP (100 μM), 2-APB (500 μM), 2′-Deoxy- N 6 -methyladenosine 3′,5′-bisphosphate (MRS2179; 500 μM) and TTX (1 μM) were from Tocris. Carbenoxolone (100 μM), PPADS (500 μM), CPA (400 μM), apyrase (grade III, 300 U ml −1 ) and ATP (50 mM) were from Sigma. TNP-ATP (100 μM) was from Jena Bioscience. Concentrations were based on initial experiments and reports [65] that effective concentrations are 100- to 1,000-fold reduced in the brain in vivo . The concentrations of MPEP [24] , [27] , carbenoxolone [11] , 2-APB [36] , PPADS [66] , CPA [50] , TTX [26] , MRS2179 (ref. 62 ), apyrase [67] , TNP-ATP [68] and ATP [26] correspond to those used in other in vivo studies. Selectivity and approximate half maximal inhibitory concentration of all inhibitors used in this study are given in Supplementary Table 2 . The dura was removed in all experiments that involved pharmacological inhibitors. In all experiments, baseline astrocytic activity was recorded before drug application. Subsequently, the silicone sealant was removed, drugs were applied topically onto the cortex for 45 min and the window was again sealed for imaging after a brief irrigation with ACSF. ATP was solubilized in ACSF and 5% Alexa 594 (Invitrogen), and delivered by microiontophoresis (MVCS, NPI electronic; 40–50 MΩ electrode impedance, −50 nA delivery current, 10 nA retaining current, 20 s). Statistical analysis Comparisons between two groups were conducted with the Mann–Whitney test. The difference between several groups was analysed using the Kruskal–Wallis test followed by Dunn’s multiple comparisons test. The Wilcoxon matched-pairs signed rank test was used for multiple measurements in the same groups. Proportions of astrocyte activity were compared with χ 2 -test. Data were analysed using Prism 6 (GraphPad, Inc.) and are expressed as mean±s.e.m. P <0.05 was accepted as statistically significant. How to cite this article: Delekate, A. et al. Metabotropic P2Y1 receptor signalling mediates astrocytic hyperactivity in vivo in an Alzheimer’s disease mouse model. Nat. Commun. 5:5422 doi: 10.1038/ncomms6422 (2014).